Visualizing short-range charge transfer at the interfaces between ferromagnetic and superconducting oxides The interplay between antagonistic superconductivity and ferromagnetism has been a interesting playground to explore the interaction between competing ground states. Although this effect in systems of conventional superconductors is better understood, the framework of the proximity effect at complex-oxide-based superconductor/ferromagnet interfaces is not so clear. The main difficulty originates from the lack of experimental tools capable of probing the interfaces directly with high spatial resolution. Here we harness cross-sectional scanning tunnelling microscopy and spectroscopy together with atomic-resolution electron microscopy to understand the buried interfaces between cuprate and manganite layers. The results show that the fundamental length scale of the electronic evolution between YBa 2 Cu 3 O 7− δ (YBCO) and La 2/3 Ca 1/3 MnO 3 (LCMO) is confined to the subnanometre range. Our findings provide a complete and direct microscopic picture of the electronic transition across the YBCO/LCMO interfaces, which is an important step towards understanding the competition between ferromagnetism and superconductivity in complex-oxide heterostructures. The interplay between superconductors (SC) and ferromagnetic (FM) metals (the so-called ‘proximity effect’) has been intensively studied for decades due to the interest in understanding the antagonistic interactions between singlet Cooper pairs with singlet alignments of spins of paired electrons, and ferromagnetism (FM) that favours parallel alignment of spins [1] . In complex-oxide-based systems composed of high-temperature superconducting YBa 2 Cu 3 O 7− δ (YBCO) and ferromagnetic La 2/3 Ca 1/3 MnO 3 (LCMO), however, these interfacial effects are still not well understood [2] , [3] . Experiments have been closely focused on the antagonism between FM- and SC-order parameters in strongly correlated systems; however, based on macroscopic physical properties, such as superconducting transition temperature and overall magnetic moment, the length scale of interactions at the boundary between the two phases is still unclear [4] , [5] , [6] , [7] , [8] , [9] , [10] , [11] , [12] , [13] , [14] . This results from a lack of a microscopic understanding of how the FM and SC phases evolve across the YBCO/LCMO interface. Although many phenomena participate at the interface (superconducting coherence, strain, magnetism, charge transfer, and so on), it becomes necessary to isolate them in order to build a proper framework of understanding. Of specific interest here is the question of interfacial charge transfer. Spatially averaged X-ray spectroscopy has demonstrated that a charge of ~0.2e − per Cu ion is transferred from Mn to Cu ions, causing an orbital reconstruction at the YBCO/LCMO interface [15] . At the same time, the length scale of the valence change measured by electron energy loss spectroscopy (EELS) between YBCO and LCMO was reported to be on the order of 4 nm, but with surprisingly opposite sign—that is, an increase in the 3 d electron count on the Mn sites, opposite to that expected from the alignment of the chemical potentials, and, more puzzling, beyond 4 nm from the interface, a reduction in the Mn 3 d electron count throughout the interior of the LCMO layer was also claimed [16] . Understanding the link between SC and charge transfer, however, requires a nanoscale-resolution probe that can spatially resolve states at the Fermi level as well as those deep in the occupied states. In this article, by utilizing the combination of cross-sectional scanning tunnelling microscopy and spectroscopy (XSTM/S) and scanning transmission electron microscopy (STEM) to study the YBCO/LCMO interface, we gain a complete picture of how the electronic and chemical structures evolve across the interface. The results demonstrate directly that the length scale of the spatial electronic evolution at the interfaces between YBCO and LCMO is <0.4 nm. The results also reveal an unexpected asymmetry of the interfacial electronic structure closely correlated with an asymmetric interface crystal structure. In short, contrary to the previously conjectured charge transfer length scales, we demonstrate that the YBCO and LCMO electronic structures are only altered within a few atomic planes from the interface, thus ruling out the long-range charge transfer scenarios. Imaging interfaces with scanning tunnelling microscopy Scanning tunneling microscopy/spectroscopy (STM/S) has excellent spatial resolution combined with the capability of simultaneously revealing the electronic local density of states (LDOS). These features of STM/S are essential for studying short-range (subnanometre) charge transfer at oxide interfaces. STM works by maintaining a constant tunnelling current at a fixed DC tip-sample bias and monitoring the tip-sample separation to measure the surface topography. At the same time, if one applies a small AC modulation to the tip bias, a lock-in technique can be utilized to measure the d I/ d V signal, which is related to the electronic LDOS at the particular bias determined by the DC voltage. Furthermore, by parking the tip at a particular location on the surface, sweeping the DC voltage and recording the d I/ d V signal, the LDOS near the Fermi energy can be measured. The spatial evolution of the d I/ d V spectra across interfaces of dissimilar materials in cross-sectional geometry can provide valuable information about the band bending/alignment. This method has been applied to study interfaces in semiconductor heterojunctions [17] , and we have recently demonstrated how this technique can be adapted to study oxide interfaces and to monitor the band bending due to the charge transfer at these oxide interfaces [18] . In order to measure the charge transfer between LCMO and YBCO, a superlattice (SL) of (LCMO(10 nm)/YBCO(10 nm)) 10 was grown on Nb-doped SrTiO 3 (001) using pulsed laser deposition [19] . (See Methods for details of sample growth.) A T c ~70 K is determined by transport measurement (see Fig. 1a ). As seen in other published studies [20] , [21] , [22] , there is a suppression of T c in the SLs (compared with the bulk value of ~91 K). A cross-sectional view of the interfaces was created by fracturing the samples in situ in the ultrahigh vacuum (UHV) chamber prior to the XSTM/S measurements [18] , [23] , [24] , [25] , [26] , [27] , [28] , [29] . 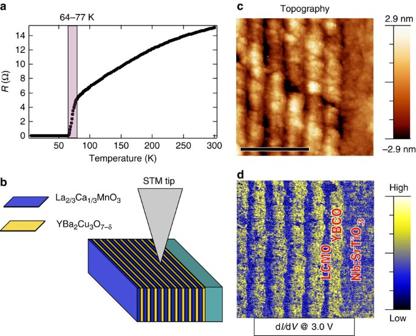Figure 1: Transport data and XSTM and dI/dVmapping at 3.0 V of the YBCO/LCMO superlattice. (a) Resistance versus temperature measurement showing a superconducting critical temperature around 70 K (64–77 K, shadowed region). (b) Schematic of cross-sectional scanning tunnelling microscopy (XSTM) on the YBCO/LCMO superlattice grown on a Nb-doped STO substrate. (c) XSTM topography and (d) dI/dVmapping at +3.0 V measured at 56 K. (c) Scale bar, 100 nm. Figure 1b shows a schematic of the geometry of the XSTM measurements in this study. Figure 1c,d shows the resulting XSTM and XSTS images recorded in the SL region at 56 K, which is below the superconducting transition temperature. The topography ( Fig. 1c ) and the STS image ( Fig. 1d ) show clear SL features. In the STS image, the YBCO exhibits bright electronic contrast compared with both the LCMO and Nb:STO regions. Note that we have previously demonstrated that the d I/ d V contrast between LCMO and Nb:STO is very similar at +3.0 V (ref. 18 ). The topography of the fractured YBCO/LCMO SLs is not atomically flat. Instead, as shown in Fig. 2 , the height variations in the averaged topography line profile are found to be on the scale of ~2 nm. As the d I/ d V contrast can be readily used to identify the different layers, by comparing the averaged topography and d I/ d V line profiles, the right and left sides of the hill in topography can thus be directly attributed to YBCO layers and LCMO layers, respectively. The main reason for the presence of the hill-valley type of topography in the cross-sectional view of the SL is still unclear, but is most probably due to the fracturing dynamics of two layers with different fracturing toughness and strain, as was discussed in Chien et al. [18] By comparing the forward and backward topography d I/ d V matching ( Fig. 2a,b ), we confirmed that the d I/ d V is free from topography-induced artefacts. Figure 1: Transport data and XSTM and d I/ d V mapping at 3.0 V of the YBCO/LCMO superlattice. ( a ) Resistance versus temperature measurement showing a superconducting critical temperature around 70 K (64–77 K, shadowed region). ( b ) Schematic of cross-sectional scanning tunnelling microscopy (XSTM) on the YBCO/LCMO superlattice grown on a Nb-doped STO substrate. ( c ) XSTM topography and ( d ) d I/ d V mapping at +3.0 V measured at 56 K. ( c ) Scale bar, 100 nm. 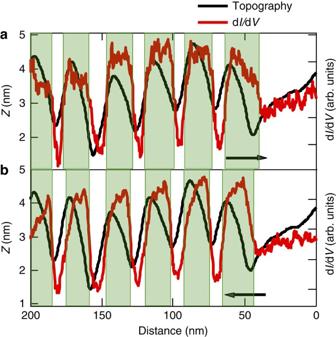Figure 2: Topography–dI/dVcorrelations in forward and backward scanning directions. Averaged line profiles of topography and dI/dVmapping for both (a) forward and (b) backward scanning directions. The line profiles are obtained by averaging along the scanning directions (arrows). Full size image Figure 2: Topography–d I/ d V correlations in forward and backward scanning directions. Averaged line profiles of topography and d I/ d V mapping for both ( a ) forward and ( b ) backward scanning directions. The line profiles are obtained by averaging along the scanning directions (arrows). Full size image Interfacial band mapping Next we turn our attention to the discussion of the electronic properties across the interfaces. We examine the spatial evolution of the LDOS by measuring a local bias-dependent d I/ d V spectrum across the YBCO/LCMO interfaces with a spatial resolution of 0.4 nm per pixel, as shown in Fig. 3a . 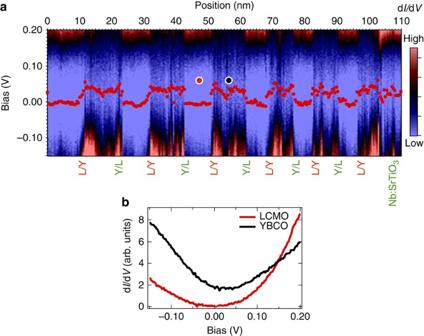Figure 3: XSTS of the YBCO/LCMO superlattice. (a) Raw line mapping of dI/dVspectra across Y/L and L/Y interfaces. Red solid marks indicate the voltage of minimum of each spectrum. It shows an asymmetry in the electronic transition at the two interfaces. The electronic transition at the Y/L interfaces is more abrupt than that at the L/Y interfaces. (b) dI/dVspectra measured in YBCO and in LCMO regions, as indicated by the black and red dots in (a), respectively. Figure 3b shows the spectra measured at the centres of an LCMO and of a YBCO layer, indicated as red and black dots in Fig. 3a . In the bulk, YBCO is a non-Fermi-liquid metallic phase above the superconducting T c [30] . On the other hand, bulk LCMO is insulating at room temperature with an energy gap of ~1.1 eV that collapses below the transition to a metallic state accompanied by FM [31] , which occurs in the SL at ~200 K. Our XSTS measurements were performed at 56 K, well below the superconducting and magnetic transition temperatures. The spectrum of LCMO ( Fig. 3b ) exhibits metallic characteristics, as indicated by the absence of an energy gap near the Fermi energy, and is symmetric with respect to zero bias, consistent with a previous study of LCMO in the metallic phase [32] . The spectrum of YBCO, on the other hand, exhibits an asymmetric shape with the minimum located at ~30 meV, in agreement with the background shape observed previously [33] . Spectroscopic features connected to the superconducting state [34] are, however, not resolved because the room-temperature tip used in this study smears out these features. Despite this k B T smearing, the LDOS probed by XSTS can provide the spatial evolution of the conduction and valence bands across the interface. Here, we use the locations of the spectra minima (indicated as red marks in Fig. 3a ) to visualize the spatial evolution of the spectra. It is also important to note that, as we are mapping surface bands, they might be altered with respect to the bulk, but, as shown below, the good correspondence between the structural and electronic interfaces, by STM and STEM, is consistent with these being closely correlated with the behaviour of the bulk bands. Figure 3: XSTS of the YBCO/LCMO superlattice. ( a ) Raw line mapping of d I/ d V spectra across Y/L and L/Y interfaces. Red solid marks indicate the voltage of minimum of each spectrum. It shows an asymmetry in the electronic transition at the two interfaces. The electronic transition at the Y/L interfaces is more abrupt than that at the L/Y interfaces. ( b ) d I/ d V spectra measured in YBCO and in LCMO regions, as indicated by the black and red dots in ( a ), respectively. Full size image A closer inspection of Fig. 3a reveals that the spectrum transition is unexpectedly asymmetric for the two types of interfaces, namely, YBCO/LCMO (Y/L) and LCMO/YBCO (L/Y). The Y/L interfaces appear to be abrupt, whereas the transitions at the L/Y interfaces are more gradual. The rough nature of the fractured surface tends to reduce the signal-to-noise ratio in the spectra. In order to gain better statistics, we perform averaging over the repeated SL cells using LCMO/YBCO half layers as the averaging block. For alignment, each interface location was determined by monitoring the d I/ d V signal at zero bias, where a drastic change could be seen in the two different materials (YBCO or LCMO). The spatial evolution of the averaged d I/ d V spectra across the two types of interfaces is given in Fig. 4a . In this d I/ d V mapping, we confirm that the evolution of the electronic properties is asymmetric across the top (L/Y) and bottom (Y/L) YBCO interfaces. The transition from LCMO to YBCO in the growth direction is abrupt, whereas the YBCO to LCMO interface is much more gradual. To quantitatively determine the electronic transition length scale, the minimum of each averaged d I/ d V spectra is determined by fitting each spectrum with parabolic function and is shown as a red dot in Fig. 4a . 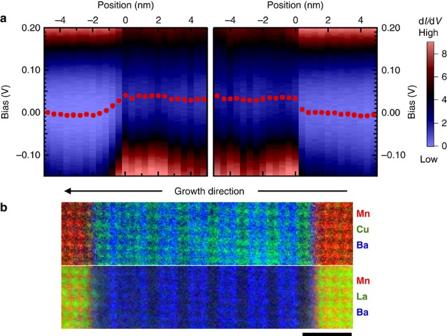Figure 4: Averaged XSTS and EELS/STEM elemental mapping of the top and bottom interfaces. (a) Spatial evolution of the averaged dI/dVspectra across the L/Y and Y/L interfaces. Red dots represent the voltage of the spectra minima. The electronic transition for YBCO/LCMO is found to be abrupt (ξY/L=0.26±0.02 nm), whereas it is broader for LCMO/YBCO (ξL/Y=0.96±0.13 nm). (b) Cross-sectional elemental mapping measured by spatially resolved EELS. Structurally asymmetric interfaces, YBCO/LCMO and LCMO/YBCO, are revealed. (b) Scale bar, 2 nm. We can further quantify this by defining a spatial decay function: Figure 4: Averaged XSTS and EELS/STEM elemental mapping of the top and bottom interfaces. ( a ) Spatial evolution of the averaged d I/ d V spectra across the L/Y and Y/L interfaces. Red dots represent the voltage of the spectra minima. The electronic transition for YBCO/LCMO is found to be abrupt ( ξ Y/L =0.26±0.02 nm), whereas it is broader for LCMO/YBCO ( ξ L/Y =0.96±0.13 nm). ( b ) Cross-sectional elemental mapping measured by spatially resolved EELS. Structurally asymmetric interfaces, YBCO/LCMO and LCMO/YBCO, are revealed. ( b ) Scale bar, 2 nm. Full size image where ɛ min ( x ) is the energy of the minimum conductance in each spectrum; ɛ 0 is the ɛ min value in YBCO at the interface, while ɛ ∞ is the value in LCMO, far from the interface; x is the distance from the interface into LCMO, while ξ is the spectrum decay length. By fitting the red dots in Fig. 4a with equation (1), ξ for both interfaces could be determined. When moving along the growth direction, the transition from LCMO into YBCO (YBCO/LCMO) is abrupt, with ξ Y/L =0.26±0.02 nm, while the transition from YBCO into LCMO (LCMO/YBCO) is by a factor of ~3 broader: ξ L/Y =0.96±0.13 nm. Though interface roughness or intermixing might also contribute to the observed spectrum evolution, these values place the upper limit for the charge transfer length scale at the YBCO/LCMO interface to, on average, less than a single YBCO unit cell along the c -axis (~1.2 nm). This length scale is remarkably similar to the order of the length scale of the suppressed magnetization (1.2±0.1 nm), but different from the transition length scale of the charge profile (~4–8 nm) observed previously [16] . Note that the surface roughness increased from less than one unit cell, for the layer close to the substrate, to ~3.5 nm, for the topmost layers, in Hoffmann et al. [16] This indicates that the interface roughness might be one origin of the discrepancy between the length scales of the charge transfer found here and in the previous report [16] . This picture is consistent with the explanation that the observed asymmetric spectra transition is due to the asymmetric chemical roughness, as will be discussed below. Two possible reasons for the observed asymmetric electronic ‘roughness’ at the interfaces are (1) an asymmetric interface stacking sequence or (2) an asymmetric interface roughness. As has been previously reported in the literature, the interfacial stacking sequences may depend on the mode of synthesis. The top/bottom interfaces of pulsed laser deposition-fabricated YBCO/LCMO SLs have asymmetric atomic plane sequences: …–BaO–CuO 2 –(La,Ca)O–MnO–… at the top and …–(La,Ca)O–MnO–BaO–CuO–BaO–CuO 2 –Y–CuO 2 –… at the bottom YBCO interface taken with respect to the growth direction [35] . In sharp contrast to this, regions of the top and bottom interfaces of sputtered LCMO/YBCO/LCMO tri-layers were reported to exhibit symmetric stacking sequences (YBCO–BaO–CuO 2 –Y–CuO 2 –BaO–MnO 2 –(La,CaO)–LCMO) by electron microscopy, even though X-ray and neutron depth profiles demonstrate that the average roughness at the LCMO/YBCO interface is larger than that of the YBCO/LCMO interface [14] , [36] . Atomic and chemical interface mapping To investigate the possible asymmetry in atomic layer stacking sequence, we have performed extensive EELS measurements in an aberration-corrected STEM at the top/bottom interfaces. With aberration-corrected STEM/EELS, atomic-resolution spectroscopic imaging of interfaces is now possible and allows an atom-column by atom-column analysis of composition and local chemical environment [37] . Using spectroscopic imaging ( Fig. 4b ), the electronically abrupt YBCO/LCMO interface is found to also be chemically abrupt with a …–BaO–CuO 2 –Y-CuO 2 –BaO–MnO 2 –(La,CaO)–… atomic layer sequence. This sequence is similar to the termination observed in sputtered YBCO/LCMO interfaces [14] . On the other hand, instead of resolving a different atomic stacking sequence, the electronically broader interface (that is, LCMO/YBCO) almost always exhibits a more disordered crystal structure. These results strongly suggest that the broader electronic interface correlates with the structurally rougher interface, while the effects from different stacking sequences are still unclear. Variations in the local chemical environment can be extracted by analysing the EELS edge fine structures. La–M, Mn–L, Ba–M, Cu–L, and O–K edge EELS spectra across the top and bottom interfaces are shown in Fig. 5a . Among them, the evolution of O–K edge spectra is of particular interest. As shown in Fig. 5c , three types of O–K edge spectra can be readily distinguished. Although there are states due to hybridization with all atoms in the system, we want to focus on the low-energy pre-peak due to hybridization with 3 d states. In Fig. 5b , we can see oxygen states due to hybridization with Mn 3 d states in LCMO as well as the apical and in-plane oxygen in YBCO (Cu–O a and Cu–O b ). The oxygen environment can be obtained by least-squares fitting to the O–K edge spectra ( Fig. 5b ). The asymmetric interface profiles can be observed in the LCMO component (the top curve in Fig. 5b ). The transition from LCMO to YBCO at the bottom interface, that is, Y/L, occurs over ~0.6 nm, which is more abrupt than the transition at the top interface (~1.2 nm). It is important to point out that the remarkably similar length scales found in EELS and STS strongly imply that the asymmetric electronic transition at both interfaces is directly coupled to the atomic roughness and that the characteristic length scale of charge transfer between YBCO and LCMO is limited to the subnanometre range. This length scale is consistent with a theoretical calculation that shows that the charge transfer in FM is roughly one to two ‘sites’ in a cubic lattice, which is ~0.4–0.8 nm (ref. 38 ). It has also been shown within the Fulde, Ferrell, Larkin and Ovchinnikov framework that the coherence length of the Cooper pairs in FM could be described by ξ F = ħν F /2 E ex , where v F is the Fermi velocity and E ex is the exchange energy in FM [1] . For LCMO, the ν F and E ex are 7.4 × 10 7 cm s −1 and 3 eV, respectively [39] ; hence, ξ F is expected to be ~0.2 nm and thus strongly supports the notion that the physics is likely confined to a subnanometre region at the interface. 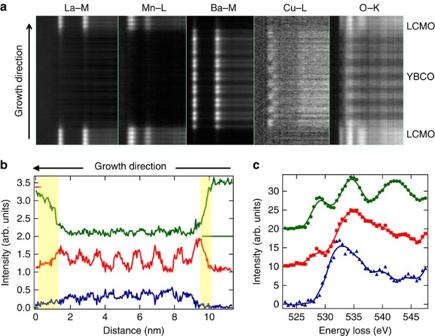Figure 5: EELS elemental mapping of the top and bottom interfaces. (a) EELS of main elements, La–M, Mn–L, Ba–M, Cu–L and O–K edges, across LCMO/YBCO/LCMO interfaces. (b) Different oxygen environment distributions obtained by least-squares fitting to the O–K edges. The EELS transition regions between LCMO and YBCO are highlighted for both interfaces. (c) Oxygen K edge spectra in different local chemical environments. In (b,c), green: LCMO; red: Cu–Oa(apical oxygen); blue: Cu–Ob(in-plane oxygen). Figure 5: EELS elemental mapping of the top and bottom interfaces. ( a ) EELS of main elements, La–M, Mn–L, Ba–M, Cu–L and O–K edges, across LCMO/YBCO/LCMO interfaces. ( b ) Different oxygen environment distributions obtained by least-squares fitting to the O–K edges. The EELS transition regions between LCMO and YBCO are highlighted for both interfaces. ( c ) Oxygen K edge spectra in different local chemical environments. In ( b , c ), green: LCMO; red: Cu–O a (apical oxygen); blue: Cu–O b (in-plane oxygen). Full size image From the combined results we conclude that for both interfaces any charge-transfer-induced band bending occurs in a subnanometre region. In other words, this result places a fundamental upper limit on the length scale for charge transfer between YBCO and LCMO. Our findings are at strong variance with the previously reported large charge-transfer length scale (~4 nm) between YBCO and LCMO by EELS [16] and theoretical SC/FM proximity effect models relying on long-range charge transfer [16] . Possible explanations for such discrepancy are as follows: (1) different sample preparation methods (high-pressure sputtering versus pulsed laser deposition (PLD)), which could result in very different stacking configurations; and (2) as described in Hoffmann et al. [16] , the interface roughness increases from submonolayer roughness close to the substrate to ~3.5 nm roughness at the topmost layers, which is similar to the charge-transfer length scale reported in the same study. Interestingly, a similar gradually increasing interfacial roughness was also observed in (LaNiO 3 ) n /(SrMnO 3 ) 2 SLs [40] . Nonetheless, the short-range charge transfer found here decisively rules out the mechanisms based on intrinsic long-range charge transfer as opposed to something structural or chemical in nature. Although proximity effects based solely on charge transfer can be excluded, it is possible that mechanisms involving coupling between charge and other degrees of freedom with longer length scale could have an important role in explaining the long-range proximity effect in YBCO/LCMO systems. Candidate mechanisms are, for examples, strain fields [41] or long-range electron–phonon coupling (consequence of long-range Coulomb forces in conjunction with a short-range orbital reconstruction at the interface) [9] . In summary, a new methodology based on the powerful combination of XSTM/S and EELS+STEM techniques has successfully been developed to directly probe the electronic and structural properties of interfaces of high- T c SC/FM SLs. The spatially resolved d I/ d V spectra provide direct evidence that the length scale for charge transfer between YBCO and LCMO has an upper limit of ~1 nm and that the spatial broadening of the electronic transition originates from rougher interfaces. In short, this result sets a fundamental upper limit on the charge-transfer length scale in the YBCO/LCMO system, ruling out a popular class of theories based on the long-range proximity effect based on charge transfer at the interfaces of YBCO and LCMO. Sample fabrication YBCO/LCMO SLs were deposited on Nb-doped SrTiO 3 (Nb:STO) (5 mm × 5 mm × 0.5 mm) by interval PLD in a layer-by-layer fashion. Fabrication of the SLs was carried out in a newly developed PLD system featuring infrared laser substrate heating and in situ monitoring via high-pressure reflection high-energy electron diffraction (HP RHEED). Stoichiometric targets of YBCO and LCMO were sequentially ablated by a KrF laser ( λ =248 nm). In the case of YBCO, the optimal conditions for 2-D growth are found to be a low laser frequency of 6–8 Hz with a dwell between the epitaxial depositions of each individual unit cell, which allowed for thermal smoothening processes. For LCMO, interval deposition with a laser frequency of 15–25 Hz proved to be the most favourable condition for a layer-by-layer growth. RHEED specular intensity oscillations are observed for both YBCO and LCMO layers, allowing for unit cell control during the construction of these SLs. The substrate temperature is continuously monitored and held at 740 °C, and an oxygen partial pressure P (O 2 )=150–200 mTorr is maintained inside the chamber throughout the deposition. Immediately after the deposition the sample is annealed at 550 °C, and the chamber is back-filled with oxygen to 500 Torr. These annealing conditions are maintained for 1 h. Scanning tunnelling microscopy The cross-sectional scanning tunnelling microscopy and spectroscopy (XSTM/S) were performed under in situ UHV fracturing with base pressure at 1.0 × 10 −10 Torr. Sample temperature could be controlled by maintaining an equilibrium of the heating/cooling power using a heater and using liquid He in the cryogenic sample stage. The cross-sectional view of the interfaces was achieved by following a controlled fracturing procedure [18] , [23] , [24] , [25] , [26] . First, the as-grown samples were diced into 1 mm × 5 mm × 0.5 mm size. A 0.5-mm notch was created by scribing from the side and the fracturing process was finished in a UHV chamber by moving the vertically mounted sample against a rigid cleaver prior to the XSTM/S measurement. The set point of the STM constant current images was set to 3.0 V and 20 pA unless specified. Electron microscopy The microstructure of the YBCO/LCMO multilayers was studied by high-angle annular dark field imaging in a FEI Tecnai F20-ST STEM. More detailed chemical composition and bonding was probed on an atomic scale using spatially resolved EELS performed on an aberration-corrected NION UltraSTEM 100, which enables two-dimensional element and valence-sensitive imaging at atomic resolution [37] . Accession Codes : The new Psychotrieae gene sequence data have been deposited in the GenBank nucleotide database under accession numbers KC480521-KC480546. How to cite this article: Chien, T. Y. et al. Visualizing short-range charge transfer at the interfaces between ferromagnetic and superconducting oxides. Nat. Commun. 4:2336 doi: 10.1038/ncomms3336 (2013).